Visible light-driven efficient overall water splitting usingp-type metal-nitride nanowire arrays Solar water splitting for hydrogen generation can be a potential source of renewable energy for the future. Here we show that efficient and stable stoichiometric dissociation of water into hydrogen and oxygen can be achieved under visible light by eradicating the potential barrier on nonpolar surfaces of indium gallium nitride nanowires through controlled p -type dopant incorporation. An apparent quantum efficiency of ∼ 12.3% is achieved for overall neutral (pH ∼ 7.0) water splitting under visible light illumination (400–475 nm). Moreover, using a double-band p- type gallium nitride/indium gallium nitride nanowire heterostructure, we show a solar-to-hydrogen conversion efficiency of ∼ 1.8% under concentrated sunlight. The dominant effect of near-surface band structure in transforming the photocatalytic performance is elucidated. The stability and efficiency of this recyclable, wafer-level nanoscale metal-nitride photocatalyst in neutral water demonstrates their potential use for large-scale solar-fuel conversion. Solar water splitting and hydrogen generation is an essential step of artificial photosynthesis for the direct conversion of solar energy into chemical fuels [1] , [2] . Among various approaches, one-step photochemical water splitting is of particular interest because of its simplicity, low-cost operation and the use of nearly neutral pH water, such as seawater for large-scale solar-fuel production [1] , [3] . It is a wireless version of photoelectrochemical water splitting in which the counter electrode is mounted on the photocatalyst surface in the form of micro/nano-electrode, that is, co-catalyst [4] . Therefore, no external bias, and hence circuitry, is required for its operation, and its efficiency is not limited by the low current conduction issue in the conventional Z-scheme process [5] . Among the currently known photocatalysts [6] , group III-nitride semiconductors, for example, indium gallium nitride (InGaN) is the only material whose energy bandgap can be tuned across nearly the entire solar spectrum and can straddle water redox potentials under ultraviolet, visible and near-infrared light irradiation [7] , [8] , thereby promising high efficiency overall water splitting under one-step photo-excitation. The extreme chemical stability of metal-nitride further demands their use as an alternative photocatalyst [9] , [10] . To date, however, the efficiency of overall water splitting on InGaN and other visible light responsive photocatalyst has remained extremely low [3] , [11] , [12] . Although an impressive solar-to-hydrogen conversion efficiency of 12.4% has been demonstrated using GaAs and p -GaInP 2 in acidic medium, such high performance cannot be sustained due to instability of the photoelectrode material, which undergoes photocorrosion under operating conditions [13] . Previously much of the research has been focused on enhancing light absorption through bandgap engineering [14] , the detrimental effect of unbalanced charge carrier extraction/collection on the efficiency of the four electron–hole water-splitting reaction has remained largely unexplored [15] , [16] . Schematically illustrated in Fig. 1 , after rapid nonadiabatic relaxation, photo-excited carriers may recombine radiatively or non-radiatively before diffusing to the near-surface region to drive redox reactions. In the emerging crystalline nanowire photocatalysts, wherein the carrier extraction efficiency is no longer diffusion-limited, the transport of spatially separated electron–hole pairs to the photocatalyst surfaces is often determined by the surface band bending [15] . Shown in the insets of Fig. 1 , the presence of an upward- (downward-) surface band bending has been commonly measured for n - ( p -) type semiconductor photocatalyst [15] , [17] . The energy barrier caused by the upward band bending repels the photo-excited electrons toward the bulk region, creating an electron depletion (hole accumulation) layer at the surface [15] , [18] . For example, the presence of ∼ 0.37 eV upward band bending can cause an electron concentration that is ∼ 20 times lower than the hole concentration on the nanowire surfaces [19] ( Supplementary Fig. 1 and Supplementary Note 1 ). This upward band bending was one of the major obstacles causing the very low ( ∼ 1.86% at 400 nm) apparent quantum efficiency (AQE) of overall water splitting on the recently reported InGaN/GaN multiband nanowire heterostructures [11] . On the other hand, the downward surface band bending of p -doped metal-nitrides creates an energy barrier for the photogenerated holes, resulting in a hole depletion (electron accumulation) at the near-surface region. This hole depletion suppresses the first-half (water oxidation) of redox reaction, which governs the rate of overall water splitting [20] . Although the presence of surface band bending is advantageous for photoelectrochemical water splitting wherein oxidation and reduction reactions take place at different electrodes, it should be minimized for photochemical water splitting to achieve balanced, efficient and stable redox reactions. Our recent study [21] suggests that by tuning the near-surface band bending on p -GaN nanowires, the quantum efficiency can be enhanced by nearly two orders of magnitude. However, it has remained unknown whether the same concept can be extended into In-containing visible light active nitrides wherein tuning of the band bending has not yet been realized owing to increased strain, defects and In phase separation along with reduced over potential to straddle the redox potential. 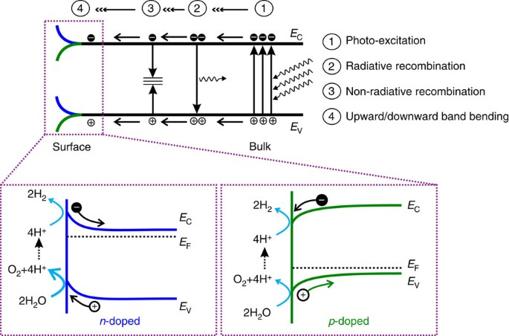Figure 1: Impact of surface band bending on the overall water splitting reaction. Schematic of carrier generation, radiative and non-radiative recombination processes. The four electron–hole water splitting mechanism is illustrated onn- (p-) doped semiconductors with upward- (downward-) surface band bending in the two bottom panels. While the oxidation reaction of water proceeds efficiently onn-doped semiconductor surface, the reduction reaction is suppressed due to the presence of upward band bending. In the case ofp-doped semiconductor, the oxidation reaction and consequently the reduction reaction are suppressed due to the presence of downward band bending at the surface. Figure 1: Impact of surface band bending on the overall water splitting reaction. Schematic of carrier generation, radiative and non-radiative recombination processes. The four electron–hole water splitting mechanism is illustrated on n - ( p -) doped semiconductors with upward- (downward-) surface band bending in the two bottom panels. While the oxidation reaction of water proceeds efficiently on n -doped semiconductor surface, the reduction reaction is suppressed due to the presence of upward band bending. In the case of p -doped semiconductor, the oxidation reaction and consequently the reduction reaction are suppressed due to the presence of downward band bending at the surface. Full size image In this context, we show that InGaN, a widely used semiconductor for solid-state lighting and power electronics, can be transformed to be an active photocatalyst under visible light irradiation by precisely engineering the surface band bending through controlled p -type Mg-dopant incorporation. The AQE of double-band p -type GaN/In 0.2 Ga 0.8 N can reach ∼ 12.3%. To the best of our knowledge, this is the highest value reported for one-step overall neutral water splitting under visible light irradiation (400–475 nm). The p -type GaN/In 0.2 Ga 0.8 N nanowire photocatalyst also exhibits a high level of stability. Growth and characterization Catalyst-free, vertically aligned InGaN nanowire arrays were grown on Si (111) substrate by radio frequency plasma-assisted molecular beam epitaxy (MBE) under nitrogen-rich conditions [22] (Methods section). Instead of direct formation of InGaN nanowires on Si substrate, a GaN nanowire template was used, which led to controlled formation of InGaN nanowires with superior structural and optical properties [23] . To minimize non-radiative recombination resulting from misfit dislocations [24] , three segments of InGaN ternary wires were incorporated along the growth direction of GaN nanowire, shown schematically in Fig. 2a . The InGaN/GaN nanowire segments were doped with divalent magnesium (Mg 2+ ) ions as p -type dopant by controlling the effusion cell temperature of Mg ( T Mg ) from 190 to 240 °C (Methods section). The GaN nanowire template was left undoped. A 45° tilted scanning electron microscopy (SEM) image ( Fig. 2b ) of as-grown InGaN nanowire arrays ( T Mg =200 °C) revealed vertically aligned nanowires, with the growth direction along the c axis. The average height is ∼ 400–600 nm, lateral sizes of the top region are ∼ 40–100 nm and the areal density is in the range of ∼ 1.5 × 10 10 cm −2 . The room temperature micro-photoluminescence (μ-PL) spectrum ( Fig. 2c ) of InGaN nanowires clearly shows a single band-to-band optical emission peak at ∼ 513 nm, which corresponds to a bandgap of 2.42 eV and average In composition of ∼ 26% (ref. 7 ). The broad emission peak reveals intra- and inter-nanowire In fluctuations, consistent with previous studies [25] . Detailed structural and elemental characterization was performed using scanning transmission electron microscopy (STEM) and energy-dispersive X-ray scanning analysis (Methods section). 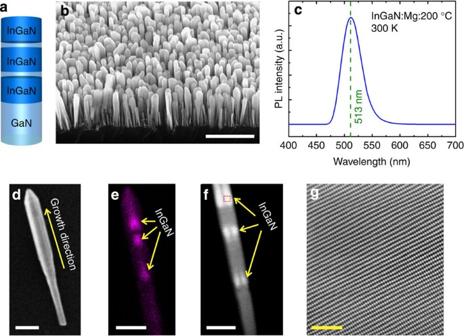Figure 2: Structural and optical properties of In0.26Ga0.74N nanowires. (a) Schematic of In0.26Ga0.74N nanowire structure showing three InGaN nanowire segments on a GaN nanowire template. (b) A 45° tilted SEM image of as-grown In0.26Ga0.74N nanowires on Si (111) substrate. Scale bar, 1 μm. (c) Room temperature μ-PL spectrum from as-grown In0.26Ga0.74N nanowires. (d) STEM-secondary electron image of a single In0.26Ga0.74N nanowire. Scale bar, 50 nm. (e) EDXS elemental (In) mapping of the In0.26Ga0.74N nanowire. Scale bar, 50 nm. (f) STEM-HAADF image of a single In0.26Ga0.74N nanowire (Fig. 2e) reveals the existence of three segments of InGaN in GaN nanowire. Scale bar, 50 nm. (g) HRSTEM-BF lattice image of the selected region inFig. 2f, illustrating lattice fringes from a defect-free single crystalline In0.26Ga0.74N nanowire. Scale bar, 2 nm. Figure 2d shows a STEM-secondary electron image of a single In 0.26 Ga 0.74 N nanowire on a carbon film. Energy-dispersive X-ray scanning (EDXS) elemental mapping ( Fig. 2e ) reveals the existence of three segments of In 0.26 Ga 0.74 N with total thickness of ∼ 80 nm within GaN nanowire. A STEM-high angle annular dark field (HAADF) image ( Fig. 2f ) further shows the atomic number contrast between In 0.26 Ga 0.74 N (brighter) and GaN (darker). No phase segregation or dislocations are observed in In 0.26 Ga 0.74 N or GaN layers, demonstrating excellent crystalline quality of the nanowires. Shown in Fig. 2g , the high crystalline quality of the In 0.26 Ga 0.74 N nanowires is further confirmed by clear lattice fringes in the high-resolution TEM image (of the selected region in Fig. 2f ). Figure 2: Structural and optical properties of In 0.26 Ga 0.74 N nanowires. ( a ) Schematic of In 0.26 Ga 0.74 N nanowire structure showing three InGaN nanowire segments on a GaN nanowire template. ( b ) A 45° tilted SEM image of as-grown In 0.26 Ga 0.74 N nanowires on Si (111) substrate. Scale bar, 1 μm. ( c ) Room temperature μ-PL spectrum from as-grown In 0.26 Ga 0.74 N nanowires. ( d ) STEM-secondary electron image of a single In 0.26 Ga 0.74 N nanowire. Scale bar, 50 nm. ( e ) EDXS elemental (In) mapping of the In 0.26 Ga 0.74 N nanowire. Scale bar, 50 nm. ( f ) STEM-HAADF image of a single In 0.26 Ga 0.74 N nanowire ( Fig. 2e ) reveals the existence of three segments of InGaN in GaN nanowire. Scale bar, 50 nm. ( g ) HRSTEM-BF lattice image of the selected region in Fig. 2f , illustrating lattice fringes from a defect-free single crystalline In 0.26 Ga 0.74 N nanowire. Scale bar, 2 nm. Full size image Surface band structure The near-surface band structure of the In 0.26 Ga 0.74 N nanowires was revealed by recording angle-resolved X-ray photoelectron spectroscopy (ARXPS) valence spectrum from the lateral nonpolar ( m -plane) surfaces of the nanowires (Methods section and Supplementary Note 2 ). 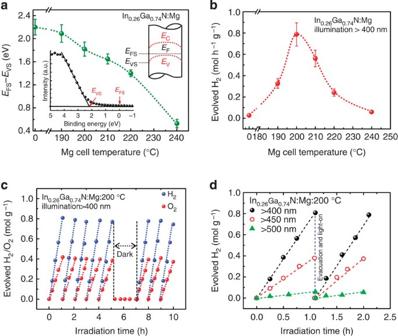Figure 3: Surface charge properties and photocatalytic activity of In0.26Ga0.74N:Mg nanowires. (a)EFS−EVSfor different Mg-doped In0.26Ga0.74N nanowire samples derived from ARXPS valence spectrum as shown in the insets. The error bars represent the accuracy of the linear extrapolation method. (b) H2evolution rate in overall neutral (pH∼7.0) water splitting for different Mg-doped In0.26Ga0.74N nanowire arrays under visible light (>400 nm). (c) The evolution of H2and O2with irradiation time from neutral (pH∼7.0) water for Mg:200 °C doped In0.26Ga0.74N nanowire arrays under dark and visible light (>400 nm) irradiation. (d) H2evolution in overall water splitting as a function of irradiation time with different long-pass filters. The experiments were performed on a∼3 cm2wafer sample (total nanowire catalyst weight∼0.32 mg) and the estimated total incident illumination intensity on the sample is 418 mW cm−2(between 400–515 nm). The dashed lines are guides to the eye. The error bar is defined by the s.d. Figure 3a shows the estimated E FS - E VS for different Mg-doped In 0.26 Ga 0.74 N samples. It is seen that E FS - E VS varies from 2.2 to 0.5 eV with increasing Mg dopant incorporation. Under relatively low Mg effusion cell temperature (low Mg flux), the dopant incorporation in the near-surface region of metal-nitride nanowire is limited by Mg desorption [21] , [26] . The surface of such In 0.26 Ga 0.74 N:Mg nanowires remains n -type, which explains the commonly measured large downward band bending on p -type InGaN surfaces [8] . The dopant incorporation can be significantly enhanced in the near-surface region with an increase in T Mg (refs 21 , 26 ). Consequently, the lateral surfaces of InGaN nanowires can be transformed from n -type to weakly p -type ( Supplementary Fig. 2 ). The extremely large tuning range ( ∼ 1.7 eV) of the surface Fermi level provides the distinct opportunity for achieving nearly flat band conditions for InGaN nanowire photocatalyst in equilibrium with water, thereby leading to very rapid diffusion of both photogenerated electrons and holes to the surfaces for high efficiency and balanced redox reactions, that was not previously possible ( Supplementary Fig. 3 and Supplementary Note 3 ). Figure 3: Surface charge properties and photocatalytic activity of In 0.26 Ga 0.74 N:Mg nanowires. ( a ) E FS − E VS for different Mg-doped In 0.26 Ga 0.74 N nanowire samples derived from ARXPS valence spectrum as shown in the insets. The error bars represent the accuracy of the linear extrapolation method. ( b ) H 2 evolution rate in overall neutral (pH ∼ 7.0) water splitting for different Mg-doped In 0.26 Ga 0.74 N nanowire arrays under visible light (>400 nm). ( c ) The evolution of H 2 and O 2 with irradiation time from neutral (pH ∼ 7.0) water for Mg:200 °C doped In 0.26 Ga 0.74 N nanowire arrays under dark and visible light (>400 nm) irradiation. ( d ) H 2 evolution in overall water splitting as a function of irradiation time with different long-pass filters. The experiments were performed on a ∼ 3 cm 2 wafer sample (total nanowire catalyst weight ∼ 0.32 mg) and the estimated total incident illumination intensity on the sample is 418 mW cm −2 (between 400–515 nm). The dashed lines are guides to the eye. The error bar is defined by the s.d. Full size image Doping-optimization Recent studies have shown that water molecules can be completely dissociatively adsorbed on nonpolar III-nitride surfaces, leading to the formation of hydroxyl species for the subsequent oxygen evolution reaction [27] . Computational and experimental analysis also suggests that the photogenerated holes on the nonpolar surfaces of GaN possess sufficient standard free energies to catalyse water oxidation [18] , [28] , [29] . A number of experimental studies have revealed that efficient water oxidation can proceed on the surface of nitrides and oxynitrides without oxidation co-catalyst [18] , [29] , [30] , [31] , [32] . To further promote H 2 evolution, Rh/Cr 2 O 3 core/shell co-catalyst [30] was photodeposited (Methods section) on In 0.26 Ga 0.74 N:Mg nanowire surfaces, wherein the Rh nanoparticles can provide more active sites for H + reduction while the Cr 2 O 3 shell layer effectively prevents any backward reaction to form water ( Supplementary Fig. 4 and Supplementary Note 4 ). The co-catalyst decorated In 0.26 Ga 0.74 N:Mg nanowire photocatalyst ( ∼ 3 cm 2 wafer sample) was subsequently used for overall neutral water (pH ∼ 7.0) splitting under visible light (>400 nm) without the presence of any sacrificial reagents (Methods section). The H 2 evolution rates in overall water splitting for different Mg-doped In 0.26 Ga 0.74 N nanowire arrays are shown in Fig. 3b . The evolution rates were derived from ∼ 6 h of water splitting for each sample. It is seen that the H 2 evolution rate first increases drastically with T Mg (increases in Mg dopant incorporation). The rate of H 2 evolution can reach ∼ 0.78 mol h −1 g −1 for the optimum Mg-doped ( T Mg =200 °C) In 0.26 Ga 0.74 N nanowire arrays, which is more than 30 times higher than that of the nominally undoped sample. The observed optimized T Mg in In 0.26 Ga 0.74 N is relatively lower than that of previously reported GaN nanowires [21] ; which is attributed to the strong dependence of Mg ionization energy on In composition and the low growth temperature of InGaN ( Supplementary Note 5 ). The significantly enhanced activity can be well explained by the tuning of the surface Fermi level and reduction in the downward surface band bending, shown in Fig. 3a , which can lead to more balanced oxidation and reduction reactions in solution ( Supplementary Fig. 3 and Supplementary Note 3 ). With further reduction in the surface band bending, however, the surface charge properties may become non-optimal for the efficient transfer of electrons and holes to the nanowire surfaces in solution, evidenced by the decrease of the overall water splitting efficiency with further increase in T Mg. Additionally, the reduction in photocatalytic activity at relatively high T Mg may be related to the deterioration of the crystal quality of the nanowires ( Supplementary Note 6 ) [33] . Figure 3c shows the evolution of H 2 and O 2 with irradiation time from neutral water splitting using the optimum ( T Mg : 200 °C) Mg-doped In 0.26 Ga 0.74 N nanowire arrays under visible light (>400 nm) irradiation. The H 2 /O 2 ratio was nearly 2:1, indicating a balanced oxidation and reduction reaction of water. The pH of water before and after reaction remained nearly the same, further confirming stoichiometric evolution of H 2 and O 2 . Repeated cycles of water splitting demonstrate the stability of In 0.26 Ga 0.74 N:Mg nanowires. While proton reduction proceeds on Rh/Cr 2 O 3 co-catalyst surface, the oxidation of water proceeds on the nonpolar sidewalls of the nanowires ( Supplementary Fig. 4e ). Note that the surface area of nonpolar In 0.26 Ga 0.74 N ( ∼ 3.0 m 2 g −1 ) nanowire sidewalls is nearly 10 times higher than the effective surface area of GaN particulate samples (0.3 m 2 g −1 ) [29] . Therefore, it is likely that the observed efficient water oxidation in the absence of oxidation co-catalyst is partly due to a high number of surface reaction sites. However, the exact mechanism of such efficient multi-step water oxidation reaction on metal-nitride surface remains unclear to date, and requires further detailed studies [20] . Our control experiment also confirms that photo-excited charge carriers in Si substrate do not take part in the photochemical reaction, which can be directly correlated to the presence of large band-offset at the Si/GaN interface and insufficient water oxidation potential of Si ( Supplementary Fig. 5 ) [34] . The wavelength dependent activity of In 0.26 Ga 0.74 N:Mg:200 °C nanowires is revealed by performing overall water splitting with different long-pass filters, shown in Fig. 3d . Significant activity was observed for excitation up to 520 nm, which is consistent with the band edge of In 0.26 Ga 0.74 N:Mg nanowires (PL peak ∼ 513 nm, Fig. 2c ). Overall water splitting on double-band nanowire heterostructures We have subsequently developed multi-stacked broadband GaN:Mg/InGaN:Mg nanowire photocatalyst, schematically shown in Fig. 4a , wherein the surface charge properties and thicknesses of the GaN and InGaN segments are separately optimized to achieve maximum efficiency in the UV and visible wavelength range, respectively (Methods section). In this case, five segments of InGaN ternary wires were incorporated along the growth direction of GaN nanowires to enhance light absorption, as shown in Fig. 4a . Shown in Fig. 4a inset, the GaN:Mg/InGaN:Mg nanowire photocatalyst can effectively function as a double-band heterostructure to efficiently harness UV and visible solar photons. The room temperature μ-PL measurement ( Fig. 4b ) reveals two band-to-band emission peaks at ∼ 364 nm and ∼ 475 nm, corresponding to the bandgap of GaN (3.4 eV) and InGaN (2.61 eV), respectively. The dual-bandgap system is adopted for better matching and utilization of solar spectrum, and to minimize the energy loss due to the rapid thermal relaxation of high-energy charge carriers [35] . The average In composition in InGaN segments is ∼ 20% (ref. 7 ). The STEM-HAADF image, as presented in Fig. 4c , clearly shows the atomic number contrast between In 0.2 Ga 0.8 N segments (brighter contrast) and GaN nanowire. The In 0.2 Ga 0.8 N total thickness is ∼ 185 nm. The EDXS elemental (In, Ga, N) mapping image of the nanowire heterostructure is illustrated in the inset of Fig. 4c . The p -type behaviour of the GaN:Mg and In 0.20 Ga 0.80 N:Mg nanowire are confirmed by open-circuit potential (OCP) measurements ( Supplementary Fig. 6 and Supplementary Note 7 ) [36] . With the incorporation of Rh/Cr 2 O 3 core/shell nanoparticles on the p -GaN/ p -In 0.20 Ga 0.80 N nanowires, overall water splitting was performed with different long-pass filters in the absence of any sacrificial reagents under 300 W Xenon lamp irradiation. The rates of H 2 and O 2 evolution are shown in Fig. 4d , which are determined from ∼ 6 h of water splitting. The H 2 and O 2 evolution rates were ∼ 3.46 mol h −1 g −1 and ∼ 1.69 mol h −1 g −1 , respectively, under full arc illumination with AM1.5G filter ( ∼ 26 suns). Bubbles of H 2 and O 2 formed due to overall neutral water splitting were clearly observed ( Fig. 4e ) upon irradiation ( Supplementary Movie 1 ). The pH of water remained the same over the course of reaction, showing unambiguous evidence of balanced reaction. The photocatalytic activity decreased with increase in wavelength, limited by the optical absorption of the nanowire catalyst. 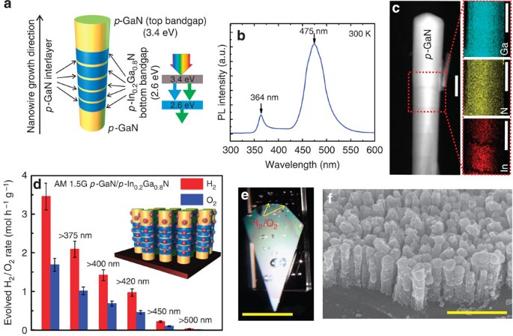Figure 4: Material properties and photochemical activity ofp-GaN/p-In0.20Ga0.8N nanowires. (a) Schematic of the double-band GaN/In0.20Ga0.8N nanowire heterostructure illustrating different layers incorporated during growth for efficient photon absorption and water-splitting reaction. Five segments of InGaN were incorporated along the growth axis of GaN nanowires. The concept of double-band photocatalyst is illustrated in the inset. (b) Room temperature μ-PL spectrum from as-grownp-GaN/p-In0.20Ga0.8N nanowire heterostructure. (c) STEM-HAADF image of a singlep-GaN/p-In0.20Ga0.8N nanowire reveals the existence of In0.20Ga0.8N segments in GaN nanowire. The inset shows EDXS elemental mapping on the selected region of thep-GaN/p-In0.20Ga0.8N nanowire, showing the distribution of In, Ga and N. Scale bar, 50 nm. (d) H2and O2evolution rates in overall water splitting with AM1.5G filter, and with different long-pass filters. Visible light activity is clearly demonstrated. The inset shows a schematic of core/shell Rh/Cr2O3nanoparticle decorated double-bandp-GaN/p-In0.20Ga0.8N nanowire photocatalyst on Si substrate. The error bar is defined by the s.d. (e) A snapshot of H2and O2gas bubble formation from neutral water under full arc illumination with AM1.5G optical filter on ap-GaN/p-In0.20Ga0.8N sample (Supplementary Movie 1). A∼3 cm2sample (active GaN/In0.2Ga0.8N catalyst weight∼0.48 mg) was glued on a microscopic glass and immersed in neutral pH water for overall water splitting. Scale bar, 2 cm. (f) SEM image of thep-GaN/p-In0.20Ga0.8N nanowire after∼6 h of water splitting, demonstrating the stability of nanowires and Rh/Cr2O3co-catalyst. Scale bar, 1 μm. Figure 4: Material properties and photochemical activity of p -GaN/ p -In 0.20 Ga 0.8 N nanowires. ( a ) Schematic of the double-band GaN/In 0.20 Ga 0.8 N nanowire heterostructure illustrating different layers incorporated during growth for efficient photon absorption and water-splitting reaction. Five segments of InGaN were incorporated along the growth axis of GaN nanowires. The concept of double-band photocatalyst is illustrated in the inset. ( b ) Room temperature μ-PL spectrum from as-grown p -GaN/ p -In 0.20 Ga 0.8 N nanowire heterostructure. ( c ) STEM-HAADF image of a single p -GaN/ p -In 0.20 Ga 0.8 N nanowire reveals the existence of In 0.20 Ga 0.8 N segments in GaN nanowire. The inset shows EDXS elemental mapping on the selected region of the p -GaN/ p -In 0.20 Ga 0.8 N nanowire, showing the distribution of In, Ga and N. Scale bar, 50 nm. ( d ) H 2 and O 2 evolution rates in overall water splitting with AM1.5G filter, and with different long-pass filters. Visible light activity is clearly demonstrated. The inset shows a schematic of core/shell Rh/Cr 2 O 3 nanoparticle decorated double-band p -GaN/ p -In 0.20 Ga 0.8 N nanowire photocatalyst on Si substrate. The error bar is defined by the s.d. ( e ) A snapshot of H 2 and O 2 gas bubble formation from neutral water under full arc illumination with AM1.5G optical filter on a p -GaN/ p -In 0.20 Ga 0.8 N sample ( Supplementary Movie 1 ). A ∼ 3 cm 2 sample (active GaN/In 0.2 Ga 0.8 N catalyst weight ∼ 0.48 mg) was glued on a microscopic glass and immersed in neutral pH water for overall water splitting. Scale bar, 2 cm. ( f ) SEM image of the p -GaN/ p -In 0.20 Ga 0.8 N nanowire after ∼ 6 h of water splitting, demonstrating the stability of nanowires and Rh/Cr 2 O 3 co-catalyst. Scale bar, 1 μm. Full size image The absorbed photon conversion efficiency (APCE) and AQE of the p -GaN/ p -In 0.2 Ga 0.8 N double-band nanowire photocatalyst are derived to be ∼ 74.5% and ∼ 20%, respectively ( Supplementary Note 8 ) in the wavelength range 200–475 nm. In the range of 400–475 nm, the APCE and AQE are estimated to be ∼ 69% and 12.3%, respectively ( Supplementary Note 8 ). Note that, taking into account light reflection and scattering, the APCE may be reduced by 10–15%. The achieved AQE of 12.3% at 400–475 nm of our photocatalyst is more than two times higher than the most efficient (AQE ∼ 5.9% at 420–440 nm) and stable visible light active photocatalyst in overall water splitting reported to date [37] . Additionally, the energy conversion efficiency (ECE) is estimated to be ∼ 7.5% under UV and visible light (incident power intensity ∼ 488 mW cm −2 for the wavelength range 200–475 nm) ( Supplementary Note 8 ), which is much higher than the recently reported values [38] , [39] for one-step overall water splitting and is comparable to that of wireless or wired water splitting device comprised of integrated photovoltaic cells [13] , [40] . Moreover, the solar-to-hydrogen (STH) conversion efficiency i.e., the ECE under full arc illumination with AM1.5G filter ( ∼ 26 suns) is estimated to be ∼ 1.8% ( Supplementary Fig. 7 and Supplementary Note 8 ), which is an order of magnitude higher than that of recently reported one-step overall water splitting photocatalyst [38] , [39] . Although the STH conversion efficiency of p -GaN/ p -In 0.2 Ga 0.8 N nanowire catalyst is lower than the recently reported ∼ 5% STH efficiency of CoO nanoparticles [41] for overall water splitting, the stability (for over 10 h) of p -GaN/ p -In 0.2 Ga 0.8 N nanowires is far better than that of CoO nanoparticles (deactivated after 1 h). The turnover number (TON), in terms of the ratio of the total amount of gas (H 2 and O 2 ) evolved per hour ( ∼ 2.47 mmol) to the amount of p -GaN/ p -In 0.2 Ga 0.8 N catalyst ( ∼ 0.48 mg), exceeded ∼ 5.15 mol h −1 g −1 under full arc illumination with AM1.5G filter. Under visible light (>400 nm) the TON is estimated to be ∼ 2.0 mol h −1 g −1 . This extremely high TON can essentially overcome the barrier for large-scale practical applications of the III-nitride nanowire photocatalyst. It is also worthwhile discussing the charge carrier separation mechanism of the present nanowire catalyst. Under nearly flat band conditions, the charge carrier separation and extraction is largely dominated by diffusion. In this study, the lateral dimensions of InGaN/GaN nanowires are in the range of 40–100 nm ( Supplementary Fig. 9 ), which is much smaller than the diffusion lengths ( ∼ 200–300 nm) of photo-excited charge carriers [8] . Our previous analysis of charge carrier transport in InGaN/GaN nanowire structures showed that ∼ 90% of the charge carriers can readily diffuse to the nanowire surface under flat band conditions [19] . Moreover, the incorporation of Rh-cocatalyst can further enhance the charge carrier separation and extraction, evidenced by a significant reduction of the PL intensity with the presence Rh on the nanowire surfaces ( Supplementary Fig. 4d ). Repeated cycles of water splitting show no degradation of the photocatalytic activity ( Supplementary Fig. 8 ). Figure 4f shows an SEM image of the p -GaN/ p -In 0.2 Ga 0.8 N nanowire photocatalyst after ∼ 6 h of overall water splitting. The p -GaN/ p -In 0.2 Ga 0.8 N nanowire and the Rh/Cr 2 O 3 co-catalysts are stable over the course of reaction. The high stability of group III-nitrides, which has also been confirmed in several other studies [10] , [42] , [43] , [44] , [45] , [46] , is ascribed to the large difference in electronegativity between group III and group V elements that can lead to the absence of surface states within the fundamental energy bandgap [47] , [48] . The achievement of efficient and stable water splitting on III-nitride photocatalyst promises viable industrial production of hydrogen by artificial photosynthesis [1] . In summary, we have shown that the concept of controlling surface band bending can be extended to InGaN nanowires by overcoming the growth challenges for achieving nearly defect-free Mg-doped InGaN nanowires. We have further demonstrated visible light-driven efficient and stable overall water splitting on metal-nitride nanowire arrays by minimizing the potential barrier at the nonpolar nanowire surfaces through precise tuning of the surface band bending. In addition, the concept of dual-bandgap scheme has been unambiguously demonstrated to enhance the efficiency. The wireless oxygen and hydrogen-evolving reactions occur in water at neutral pH and with sunlight as the only energy input, as is in the natural photosynthetic process. The STH conversion efficiency can further be improved by utilizing multiband InGaN nanowire photocatalysts with high (up to ∼ 50%) indium compositions to enable spontaneous overall water splitting under deep-visible and near-infrared light irradiation. However, a number of growth-related issues need to be addressed, including indium phase separation, indium surface segregation and the formation of misfit dislocations due to the large lattice mismatch ( ∼ 11%) between InN and GaN [8] . MBE growth The vertically aligned InGaN nanowires were grown on Si (111) substrate by radio frequency plasma-assisted MBE under nitrogen-rich conditions without using any foreign catalyst. Before loading into the MBE chamber, the Si (111) substrate was rinsed with acetone and methanol to remove organic contaminants and subsequently with 10% hydrofluoric acid to remove native oxide. In situ oxide desorption was performed at ∼ 770 °C before the growth initiation until the formation of a clean Si (111) 7 × 7 reconstructed surface was confirmed by reflection high-energy electron diffraction. A thin (approximately one monolayer) gallium (Ga) seeding layer was in situ deposited, which promotes the nucleation of nanowires. Thermal effusion cells were used for Ga, In and Mg. Nitrogen radicals were supplied from a radio frequency plasma source. The growth parameters include nitrogen flow rate of 1.0 standard cubic centimeters per minute (s.c.c.m. ), a forward plasma power of ∼ 350 W, and a Ga beam equivalent pressure (BEP) of ∼ 6 × 10 −8 Torr. The In BEP was ∼ 8 × 10 −8 Torr. The Mg effusion cell temperature was varied from 190 to 300 °C, which corresponds to Mg BEP of ∼ 1.0 × 10 −11 to ∼ 7.3 × 10 −9 Torr. The estimated Mg concentration at Mg cell temperatures of 200, 230 and 250 °C is ∼ 2.8 × 10 18 cm −3 , ∼ 4.1 × 10 19 cm −3 and ∼ 1.3 × 10 20 cm −3 , respectively; which were measured from secondary ion mass spectroscopy (SIMS) analysis on Mg-doped GaN epilayers grown under similar growth conditions (that is, similar Mg cell temperature). The growth temperature for GaN was ∼ 750 °C. The growth temperature for InGaN was in the range of 640 to 680 °C. For the growth of multi-stacked broadband GaN:Mg/InGaN:Mg nanowire photocatalyst ( Fig. 4a ), the five InGaN segments were doped at T Mg =200 °C and the top GaN segment was doped at T Mg =270 °C ( Supplementary Note 8 ). Micro-photoluminescence The μ-PL measurement was performed with either a 405-nm laser or a 325-nm He-Cd laser (Kimmon Koha) as excitation source. The laser beam was focused on the sample through a × 60 objective, with a circular beam size of ∼ 5 μm. The emitted light was collected by the same objective and spectrally resolved by a high-resolution spectrometer and detected by a photomultiplier tube. Scanning transmission electron microscopy For STEM-secondary electron, STEM-BF and STEM-HAADF imaging, a Hitachi HD2700 Cs-corrected STEM was used with a cold field emitter operated at 200 kV and with an electron beam diameter of ∼ 0.1 nm. STEM EDS analysis was performed using a 60 mm 2 silicon drift detector from Bruker. A radial difference filter is used to process Fig. 2g . Photodeposition of co-catalyst The nanowires were decorated with Rh/Cr 2 O 3 core/shell nanoparticles using a two-step photodeposition process from liquid precursors. In the first step, Rh particles were photodeposited from sodium hexachlororhodate (III) (Na 3 RhCl 6 , Sigma-Aldrich) precursor in the presence of 20% methanol in water. In the second step, the Cr 2 O 3 was photodeposited from potassium chromate (K 2 CrO 4 , Sigma-Aldrich) precursor in the presence of 20% methanol in water. Our previous X-ray photoelectron spectroscopy analysis suggests that the co-catalysts form a Rh metallic core, a mixed Rh–Cr oxide interfacial layer and a Cr 2 O 3 shell on the nanowire surface [11] . Angle-resolved X-ray photoelectron spectroscopy Thermo Fisher Scientific K-Alpha XPS system equipped with a monochromatic Al-Kα X-ray source ( hυ =1,486.6 eV) and 180° double focusing hemispherical analyser was used for the analysis. The analysis chamber pressure was ∼ 10 −8 Torr. The X-ray source is located at 60° with the surface normal to excite the nonpolar surfaces of nanowire arrays. The binding energies were calibrated with both Au 4f (84.0 eV) and C 1s (285.0 eV) peaks. The E FS − E VS was estimated for each sample from ARXPS valence band spectrum. The intersection between the linear extrapolation of the valence band leading edge and the baseline ( Fig. 3a inset) indicates the position of surface valence band ( E VS ) with respect to the surface Fermi level ( E FS , binding energy=0 eV) [49] . Photocatalytic reaction The overall water splitting reaction was performed by adopting a 300 W Xenon lamp (Cermax, PE300BUV) as an outer irradiation ( Supplementary Fig. 10 ) source. The sample was placed with a homemade polytetrafluoroethylene holder in a Pyrex chamber with a quartz lid. Distilled water was purged with Ar for 20–30 min before each experiment. The chamber was then evacuated. A vacuum-tight syringe was used for sampling the reaction evolved gases (H 2 and O 2 ) and analysed by a gas chromatograph (Shimadzu GC-8A) equipped with thermal conductivity detector and high-purity Ar carrier gas. The reaction chamber was air cooled, and the average water temperature during the experiment was nearly 45 °C. The experimental error in the evolution of H 2 and O 2 is estimated to be ∼ 10% due to manual sampling of the evolved gases and leakage through the septum. How to cite this article: Kibria, M. G. et al. Visible light-driven efficient overall water splitting using p -type metal-nitride nanowire arrays. Nat. Commun. 6:6797 doi: 10.1038/ncomms7797 (2015).